Mycobacterium tuberculosisacquires iron by cell-surface sequestration and internalization of human holo-transferrin Mycobacterium tuberculosis ( M.tb ), which requires iron for survival, acquires this element by synthesizing iron-binding molecules known as siderophores and by recruiting a host iron-transport protein, transferrin, to the phagosome. The siderophores extract iron from transferrin and transport it into the bacterium. Here we describe an additional mechanism for iron acquisition, consisting of an M.tb protein that drives transport of human holo-transferrin into M.tb cells. The pathogenic strain M.tb H37Rv expresses several proteins that can bind human holo-transferrin. One of these proteins is the glycolytic enzyme glyceraldehyde-3-phosphate dehydrogenase (GAPDH, Rv1436), which is present on the surface of M.tb and its relative Mycobacterium smegmatis . Overexpression of GAPDH results in increased transferrin binding to M.tb cells and iron uptake. Human transferrin is internalized across the mycobacterial cell wall in a GAPDH-dependent manner within infected macrophages. M ycobacterium tuberculosis (M.tb) is an intracellular pathogen that persists within the host cell phagosome for extended periods and a regular supply of iron is essential for its survival. To acquire iron, mycobacteria synthesize iron-chelating molecules known as siderophores. M.tb utilizes both membrane-associated mycobactins and secreted carboxymycobactins to sequester host iron [1] , [2] , [3] . In addition, this pathogen also acquires iron from haem [4] ; intracellular M.tb are known to actively recruit host iron carrier proteins transferrin and lactoferrin to the phagosomal compartment [5] , [6] , [7] , [8] . It is reported that carboxymycobactins remove iron from transferrin in the phagosome, while mycobactins present in the bacterial membrane transport this iron into the bacterial cytoplasm [9] , [10] . Carboxymycobactin also delivers iron by a mycobactin-independent mechanism using the IrtAB transporter [11] . However, the detailed process by which transferrin iron is released and whether other mycobacterial components are involved in the process remain unknown [12] . The absence of mycobactin in M.tb- infected tissues suggests that alternate iron acquisition mechanisms may exist in vivo [13] . The same study demonstrated that at pH 6.2, the presence of host proteins transferrin and lactoferrin promoted the growth of M. paratuberculosis mycobactin auxotrophs in culture. This aspect cannot be explained by the simple dissociation of bound iron from transferrin and lactoferrin, which is known to occur maximally at pH 5.5-4.0 (ref. 13 ). Another recent study demonstrates that the recombinant BCG( mbtB )30 strain which is unable to synthesize both mycobactin and carboxymycobactin retains the ability to multiply and survive within macrophages over the initial days of infection [14] . The importance of transferrin in mycobacterial iron acquisition is also evident from studies demonstrating that intraphagosomal M.tb siderophore knockout strains retained the ability to recruit and acquire iron by utilizing transferrin [5] , [14] , [15] . Other studies have demonstrated that iron-saturated transferrin promotes the replication of M. avium within the phagosome [15] . Elevated serum iron and high levels of iron-saturated transferrin are known to have a strong correlation with the exacerbation of tuberculosis in both mouse models and patient studies [3] , [16] , [17] , [18] , [19] , [20] . Several pathogens including Staphylococcus aureus , S. epidermidis, N. meningitidis, N. gonorrhoeae, H. influenza and others are known to acquire iron by the direct binding of transferrin on the cell surface [21] , [22] , [23] , [24] . However, no in vivo or in vitro studies have ever identified the existence of transferrin-binding proteins on the surface of M.tb. Here we report the presence of several proteins that are capable of sequestering transferrin at the bacterial cell surface. Transferrin-iron acquisition by this pathway is independent of siderophores. Instead, transferrin-associated iron is obtained by the trafficking and internalization of the host protein across the bacterial cell wall, a mechanism not previously reported for M.tb . This pathway is utilized during the infection of macrophages by intracellular bacilli and is relevant in understanding the fundamental mechanisms of iron acquisition in M.tb. Transferrin binds to M.tb Intact M.tb H37Ra cells were observed to bind Transferrin-Alexa 647 (Tf-A647). The specificity of binding was confirmed by the inhibition of labelling in the presence of 200-fold excess of unlabelled transferrin ( P < 0.05 , determined by Student’s t -test; Fig. 1a ). The surface of intact M.tb H37Ra was also decorated with transferrin-conjugated gold particles as visualized by Transmission Electron Microscope (TEM; Fig. 1b , Supplementary Fig. 1a–e ) as compared with controls ( Fig. 1c ). 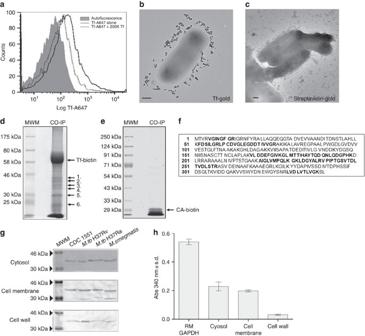Figure 1:M. tuberculosisexpresses cell surface transferrin binding proteins including GAPDH. (a) FACS analysis indicates specific binding of Tf-A647, (P<0.05,estimated by Student’st-test, experiments were repeated thrice (n=3), 104cells were analysed each time. (b) Transferrin-conjugated gold particles localize on the surface of intactM.tbH37Ra (see alsoSupplementary Fig. 1a–e), scale bar, 0.2 μm. (c) No surface labelling is observed in controls (Streptavidin-gold conjugate), scale bar, 0.2 μm. Multiple fields were analysed with each sample, representative images are shown. (d,e) Co-immunoprecipitation ofM.tbH37Rv membrane proteins using (d) transferrin and (e) carbonic anhydrase (nonspecific negatively charged protein control). Prestained molecular weight markers were run alongside, arrows indicate proteins selected for further analysis. (f) Peptide mass fingerprinting analysis of 40 kDa protein (GAPDH) fromM.tbH37Rv membrane (identified peptides are indicated in bold). (g) Localization of GAPDH in the cytoplasm, membrane and cell wall fractions ofM.tbCDC1551, H37Rv,M.tbH37Ra andM. smegmatis.(see alsoSupplementary Fig. 1f,gandSupplementary Fig. 6a–c). (h) GAPDH enzyme activity in cytosol, cell membrane and cell wall fractions ofM.tbH37Rv. Results are expressed as absorbance at 340 nm±s.d. (n=3; that is, three independent batches) after 10 min incubation. Rabbit muscle GAPDH (RM-GAPDH) was used as a positive control; negative control values (without specific substrate G-3-P) have been subtracted for each sample. Figure 1: M. tuberculosis expresses cell surface transferrin binding proteins including GAPDH. ( a ) FACS analysis indicates specific binding of Tf-A647, ( P < 0.05, estimated by Student’s t -test, experiments were repeated thrice ( n =3), 10 4 cells were analysed each time. ( b ) Transferrin-conjugated gold particles localize on the surface of intact M.tb H37Ra (see also Supplementary Fig. 1a–e ), scale bar, 0.2 μm. ( c ) No surface labelling is observed in controls (Streptavidin-gold conjugate), scale bar, 0.2 μm. Multiple fields were analysed with each sample, representative images are shown. ( d , e ) Co-immunoprecipitation of M.tb H37Rv membrane proteins using ( d ) transferrin and ( e ) carbonic anhydrase (nonspecific negatively charged protein control). Prestained molecular weight markers were run alongside, arrows indicate proteins selected for further analysis. ( f ) Peptide mass fingerprinting analysis of 40 kDa protein (GAPDH) from M.tb H37Rv membrane (identified peptides are indicated in bold). ( g ) Localization of GAPDH in the cytoplasm, membrane and cell wall fractions of M.tb CDC1551, H37Rv, M.tb H37Ra and M. smegmatis. (see also Supplementary Fig. 1f,g and Supplementary Fig. 6a–c ). ( h ) GAPDH enzyme activity in cytosol, cell membrane and cell wall fractions of M.tb H37Rv. Results are expressed as absorbance at 340 nm±s.d. ( n =3; that is, three independent batches) after 10 min incubation. Rabbit muscle GAPDH (RM-GAPDH) was used as a positive control; negative control values (without specific substrate G-3-P) have been subtracted for each sample. Full size image Co-immunoprecipitation and peptide mass fingerprinting Co-immunoprecipitation from M.tb H37Rv cell membrane fraction to determine the identity of transferrin-binding protein(s) indicated the presence of several proteins in the range of 25–40 kDa ( Fig. 1d ). Pull-down using carbonic anhydrase (a negatively charged protein, as a nonspecific control) did not reveal the presence of any interacting proteins ( Fig. 1e ). This indicates that the proteins identified by co-immunoprecipitation with transferrin were specific. Peptide mass fingerprinting (PMF) of the most prominent proteins identified these as iron-regulated elongation factor tu (Rv0685, 25% coverage, molecular weight search (MOWSE ) score 107), L -Lactate dehydrogenase (Rv1872c; 38% coverage, MOWSE score 83), acyl-carrier protein desaturase (Rv0824c; 16% coverage, MOWSE score 166), 50S ribosomal protein L2 (Rv0704; 46% coverage, MOWSE score 100), 50S ribosomal protein L1 (Rv0641; 37% coverage, MOWSE score 269) and GAPDH (Rv1436; 32% coverage, MOWSE score 552; Table 1 , Fig. 1f ). The MOWSE score is a protein identification programme that recognizes the relative abundance of peptides of a given length. This programme calculates the probability that the observed match between the experimental data set and each sequence database entry is a chance event, the match with the lowest probability is reported as the best match [25] . Table 1 M.tb proteins co-immunoprecipitated by holo-transferrin. Full size table We selected GAPDH for further analysis because: (i) GAPDH has recently been identified as a transferrin receptor in macrophages and numerous other cell types [26] , [27] , [28] , (ii) the highly conserved nature of the protein and (iii) its role as a virulence factor [29] , [30] , [31] , [32] . Localization of GAPDH in different cellular fractions A peptide sequence from amino acid 59–100 was used to raise a rabbit polyclonal antibody against M.tb GAPDH. The antibody detected a prominent ~40 kDa protein in M.tb and M. smegmatis whole-cell lysates but did not detect GAPDH from other microorganisms or mammalian cells, indicating its specificity for mycobacterial GAPDH ( Supplementary Figs 1f and 6a ). GAPDH was found to be present in the cytosol, cell membrane and cell wall fractions of M.tb H37Ra, H37Rv and CDC1551, and in M. smegmatis ( Fig. 1g and Supplementary Fig. 6b ). The M.tb H37Ra fractions were prepared in our laboratory using standard methods and the purity of fractions was confirmed by fraction-specific antibodies ( Supplementary Figs 1g and 6c ). M.tb GAPDH has previously been detected on the cell surface as a receptor for EGF [33] . An additional faint band of ~30 kDa was detected in cell membrane fractions of all strains ( Fig. 1g ) which was also identified as GAPDH based on PMF results (47% coverage, MOWSE score 129), suggesting the presence of a proteolytically cleaved fragment ( Supplementary Fig. 1h ). Other investigators have also reported a variation in the molecular weight of GAPDH. Proteomic two-dimensional analysis of M.tb H37Rv supernatants has revealed the presence of GAPDH with a spread of molecular weights and a variation of almost 10 kDa has also been reported in GAPDH of mammalian origin (according to data available at the Proteome two-dimensional-PAGE Database, http://web.mpiib-berlin.mpg.de/cgi-bin/pdbs/2d-page/extern/index.cgi ). Enzymatic activity of cell fractions GAPDH specifically catalyses the reversible oxidative phosphorylation of glyceraldehyde-3-phosphate (G-3-P) to 1, 3-bis phosphoglycerate coupled with reduction of NAD + to NADH. Enzyme assay confirmed that GAPDH present in the cytosolic, cell membrane and cell wall of M.tb H37Rv was functionally active ( Fig. 1h ). Interaction of GAPDH and transferrin on M.tb cell surface The interaction of transferrin and GAPDH was checked by co-immunoprecipitation. Transferrin was observed to interact with mycobacterial GAPDH from all three cellular fractions ( Fig. 2a and Supplementary Fig. 6d ). 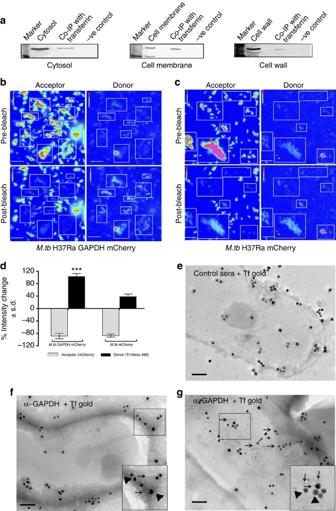Figure 2: Transferrin interacts with GAPDH bothin vitroandin vivo. (a) Biotinylated transferrin co-immunoprecipitates GAPDH from cytosolic, membrane and cell wall fractions ofM.tbH37Rv (see alsoSupplementary Fig. 6d). (b) Acceptor photobleaching FRET analysis of the GAPDH–transferrin interaction on the surface ofM.tbH37Ra cells. An increase in donor (Tf-A488) signal is observed upon bleaching of acceptor (GAPDH-mCh). Boxes indicate clusters of cells that were bleached for the experiment. (c) Control experiment usingM.tbH37Ra expressing mCh alone. FRET experiments were repeated twice with multiple fields analysed each time, representative images are shown (see alsoSupplementary Fig. 2). Scale bar, 10 μm, blue to red intensity bar is in the range 0–4096. (d) Quantitative analysis of FRET signal. Three different fields were analysed for each experiment, four regions from each field were randomly selected, % intensity change±s.d. of the donor and acceptor signals after photobleaching GAPDH-mCh or mCh was determined using ImageJ software. The % intensity change of Tf-A488 signal was significantly higher in cells expressing GAPDH-mCh as compared with cells expressing mCh alone (***P<0.0001, Student’st-test;n=12, three different fields with four regions of interest from each field). Colocalization of GAPDH and transferrin by Immunogold Transmission Electron Microscopy onM.tbH37Ra GAPDH-mCh expressing strain. (e) Cells were labelled with 1:100 dilution of rabbit pre-immune sera as control followed by secondary antibody conjugated with 5-nm gold particles. (f,g) GAPDH was detected using 1:100 polyclonal rabbit α-GAPDH followed by secondary antibody conjugated with 5-nm gold particles, scale bar, 100 nm. All cells were simultaneously labelled with transferrin-gold conjugate. Inset: Magnified image of highlighted area showing colocalization of GAPDH and transferrin. Arrows indicate 5-nm particles (GAPDH); arrowheads indicate the presence of transferrin-gold. Experiments were repeated four times, representative fields are shown. Figure 2: Transferrin interacts with GAPDH both in vitro and in vivo. ( a ) Biotinylated transferrin co-immunoprecipitates GAPDH from cytosolic, membrane and cell wall fractions of M.tb H37Rv (see also Supplementary Fig. 6d ). ( b ) Acceptor photobleaching FRET analysis of the GAPDH–transferrin interaction on the surface of M.tb H37Ra cells. An increase in donor (Tf-A488) signal is observed upon bleaching of acceptor (GAPDH-mCh). Boxes indicate clusters of cells that were bleached for the experiment. ( c ) Control experiment using M.tb H37Ra expressing mCh alone. FRET experiments were repeated twice with multiple fields analysed each time, representative images are shown (see also Supplementary Fig. 2 ). Scale bar, 10 μm, blue to red intensity bar is in the range 0–4096. ( d ) Quantitative analysis of FRET signal. Three different fields were analysed for each experiment, four regions from each field were randomly selected, % intensity change±s.d. of the donor and acceptor signals after photobleaching GAPDH-mCh or mCh was determined using ImageJ software. The % intensity change of Tf-A488 signal was significantly higher in cells expressing GAPDH-mCh as compared with cells expressing mCh alone (*** P < 0.0001 , Student’s t -test; n =12, three different fields with four regions of interest from each field). Colocalization of GAPDH and transferrin by Immunogold Transmission Electron Microscopy on M.tb H37Ra GAPDH-mCh expressing strain. ( e ) Cells were labelled with 1:100 dilution of rabbit pre-immune sera as control followed by secondary antibody conjugated with 5-nm gold particles. ( f , g ) GAPDH was detected using 1:100 polyclonal rabbit α-GAPDH followed by secondary antibody conjugated with 5-nm gold particles, scale bar, 100 nm. All cells were simultaneously labelled with transferrin-gold conjugate. Inset: Magnified image of highlighted area showing colocalization of GAPDH and transferrin. Arrows indicate 5-nm particles (GAPDH); arrowheads indicate the presence of transferrin-gold. Experiments were repeated four times, representative fields are shown. Full size image Having established that this interaction occurs in the pathogenic strain, we used M.tb H37Ra as a model system to further define whether this is a possible route for transferrin-associated iron uptake. To confirm the interaction between cell surface GAPDH and transferrin, we carried out acceptor photobleaching Förster resonance energy transfer (FRET) analysis [34] using M.tb H37Ra cells expressing GAPDH mCherry (GAPDH-mCh) or controls expressing mCherry (mCh) alone. A significant increase in donor (Tf-A488) fluorescence intensity was observed upon photobleaching of the acceptor (mCh) in strains expressing GAPDH-mCh ( Fig. 2b,d ) as compared with control cells expressing mCh alone ( Fig. 2c,d ). These results indicate the presence of a significant FRET signal as would be expected in the case of a GAPDH–transferrin interaction on bacteria. The occurrence of FRET indicates that the two interacting partners are at a proximity of 1–10 nm (ref. 34 ). Immunogold TEM further demonstrated the colocalization of GAPDH and transferrin-conjugated gold particles on the surface of intact M.tb H37Ra GAPDH-mCh cells ( Fig. 2f,g ). Controls labelled with pre-immune sera showed the presence of Tf-gold particles alone ( Fig. 2e ). Together these results suggest that transferrin interacts with GAPDH on the surface of intact bacilli. Iron depletion enhances surface GAPDH levels and Tf binding Under conditions of iron depletion, a twofold increase in GAPDH expression and a threefold increase of transferrin binding was evident on the surface of M.tb H37Ra suggesting that both surface GAPDH expression and transferrin binding are sensitive to iron levels ( Fig. 3a ). 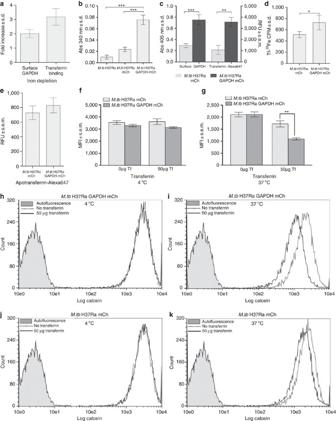Figure 3:M.tbGAPDH surface expression is sensitive to iron and is involved in iron acquisition from holo-transferrin. (a) Iron depletion caused an enhanced expression of cell surface GAPDH(P<0.005)and transferrin binding(P<0.005)onM.tbH37Ra cells. Data are plotted as fold increase±s.d., as compared with controls. (b) Enhanced cell surface GAPDH activity (ectoenzyme activity) onM.tbH37Ra cells expressing GAPDH-mCh as compared with untransformed cells (***P<0.0001) or cells expressing only mCh (***P<0.0001). Results are expressed as absorbance at 340 nm±s.d. (c) Enhanced GAPDH was detected on the surface ofM.tbH37Ra GAPDH-mCh as compared with cells expressing mCh alone (***P<0.0001, by the ELISA method using intact cells. A correlated increase of Tf-A647 binding was evident inM.tbH37Ra GAPDH-mCh as compared with controls (**P<0.005). (d)M.tbH37Ra GAPDH-mCh cells acquire significantly higher levels of55Fe from radiolabelled transferrin as compared with controls (*P<0.05). Experiments were done in duplicates and repeated twice (n=4), statistical analysis was done using Student'st-test. (e) Binding of apotransferrin does not differ significantly betweenM.tbH37Ra GAPDH-mCh and mCh strains, results are expressed as RFU±s.e.m. (f) The uptake of transferrin iron as measured by calcein-quenching assay is minimal at 4 °C for bothM.tbH37Ra GAPDH-mCh and mCh strains. (g) At 37 °C, iron uptake is significantly enhanced in theM.tbH37Ra GAPDH-mCh sample as compared with the control (**P<0.005, n=3). Data are plotted as MFI± s.e.m. (h–k).M.tbH37Ra cells expressing GAPDH-mCh (h,i) or mCh only (j,k) were stained with calcein. The quenching of fluorescence indicating iron uptake was measured at 4 °C (h,j) or 37 °C (i,k) in the absence or presence of 50 μg human holo-transferrin; unstained cells (grey area) for reference. Cells expressing GAPDH-mCh showed a significant decrease in fluorescence in the presence of transferrin at 37 °C as compared with cells expressing mCh alone. The uptake of transferrin-iron was higher at 37 °C than 4 °C in GAPDH-mCh expressing cells (P<0.005; see alsoSupplementary Fig. 3a,b). Data from 104cells per assay were acquired. For (a–c,e–k), experiments were done in duplicates and repeated thrice (n=3), statistical analysis was done using Student’st-test. Figure 3: M.tb GAPDH surface expression is sensitive to iron and is involved in iron acquisition from holo-transferrin. ( a ) Iron depletion caused an enhanced expression of cell surface GAPDH (P < 0.005) and transferrin binding (P < 0.005) on M.tb H37Ra cells. Data are plotted as fold increase±s.d., as compared with controls. ( b ) Enhanced cell surface GAPDH activity (ectoenzyme activity) on M.tb H37Ra cells expressing GAPDH-mCh as compared with untransformed cells (*** P <0.0001) or cells expressing only mCh (*** P <0.0001). Results are expressed as absorbance at 340 nm±s.d. ( c ) Enhanced GAPDH was detected on the surface of M.tb H37Ra GAPDH-mCh as compared with cells expressing mCh alone (*** P < 0.0001 , by the ELISA method using intact cells. A correlated increase of Tf-A647 binding was evident in M.tb H37Ra GAPDH-mCh as compared with controls (** P < 0.005 ). ( d ) M.tb H37Ra GAPDH-mCh cells acquire significantly higher levels of 55 Fe from radiolabelled transferrin as compared with controls (* P < 0.05 ). Experiments were done in duplicates and repeated twice ( n =4), statistical analysis was done using Student's t -test. ( e ) Binding of apotransferrin does not differ significantly between M.tb H37Ra GAPDH-mCh and mCh strains, results are expressed as RFU±s.e.m. ( f ) The uptake of transferrin iron as measured by calcein-quenching assay is minimal at 4 °C for both M.tb H37Ra GAPDH-mCh and mCh strains. ( g ) At 37 °C, iron uptake is significantly enhanced in the M.tb H37Ra GAPDH-mCh sample as compared with the control (** P < 0.005, n =3). Data are plotted as MFI± s.e.m. ( h – k ). M.tb H37Ra cells expressing GAPDH-mCh ( h , i ) or mCh only ( j , k ) were stained with calcein. The quenching of fluorescence indicating iron uptake was measured at 4 °C ( h , j ) or 37 °C ( i , k ) in the absence or presence of 50 μg human holo-transferrin; unstained cells (grey area) for reference. Cells expressing GAPDH-mCh showed a significant decrease in fluorescence in the presence of transferrin at 37 °C as compared with cells expressing mCh alone. The uptake of transferrin-iron was higher at 37 °C than 4 °C in GAPDH-mCh expressing cells ( P < 0.005 ; see also Supplementary Fig. 3a,b ). Data from 10 4 cells per assay were acquired. For ( a – c , e – k ), experiments were done in duplicates and repeated thrice ( n =3), statistical analysis was done using Student’s t -test. Full size image Enhanced surface GAPDH results in increased Tf iron uptake The cell surface GAPDH enzyme activity was assessed on M.tb H37Ra cells transformed with either mCh or GAPDH-mCh. As expected cells overexpressing GAPDH-mCh showed significantly higher ectoenzyme activity as compared with untransformed controls or mCh transformed cells ( Fig. 3b ). To assess whether this enhanced GAPDH surface expression corresponds with an increase in transferrin binding, transformed cells were evaluated for cell surface GAPDH expression and transferrin binding by whole-cell enzyme-linked immunosorbent assay (ELISA). GAPDH-mCh transformed cells demonstrated significantly higher levels of surface GAPDH along with elevated Tf-A647 binding as compared with cells expressing mCh alone ( Fig. 3c ). Enhanced GAPDH expression also correlated to a greater uptake of transferrin-associated iron by these cells as indicated by the uptake of Tf- 55 Fe in 3 h ( Fig. 3d ). To confirm whether this interaction is specific to holo-transferrin alone, both mCh and GAPDH-mCh cells were incubated with Apo-Tf-A647. No significant difference was observed between the two strains ( Fig. 3e ). To further confirm whether GAPDH enhances iron acquisition via transferrin, a calcein-quenching assay was established ( Supplementary Fig. 3a,b ). M.tb H37Ra cells expressing GAPDH-mCh or mCh were pre-labelled with calcein, followed by incubation in the absence or presence of human holo-transferrin at either 4 °C ( Fig. 3f ) or 37 °C ( Fig. 3g ). At 37 °C in the presence of transferrin, a significantly greater quenching of calcein fluorescence signal was observed in GAPDH-mCh cells as compared with those expressing mCh alone ( P <0.005 using Student’s t -test) ( Fig. 3g,i,k ). The comparatively small decrease in signal observed with mCh cells ( Fig. 3k ) can be attributed to the inherent GAPDH present on the surface of these cells. Both strains demonstrated no change in fluorescence of controls in the absence of transferrin or when incubated with transferrin at 4 °C ( Fig. 3f,h,j ). Transferrin-mediated iron uptake in M. smegmatis Δesx-3 strain GAPDH was also identified in various fractions of M. smegmatis . To assess whether (i) transferrin-mediated uptake exists across mycobacterial species and (ii) whether mycobactin is essential for iron uptake from transferrin, we utilized the M. smegmatis Δesx-3 that lacks the esx-3 secretion system and is therefore incapable of mycobactin-mediated iron uptake [35] . M. smegmatis wild-type and M. smegmatis Δesx-3 strains demonstrated no difference in binding of transferrin ( Supplementary Fig. 3c ) and both acquired comparable levels of transferrin iron within 1 h ( Supplementary Fig. 3d–f ). Affinity analysis of GAPDH-Tf interaction The interaction of rGAPDH and transferrin was first confirmed by far western blot ( Supplementary Fig. 4a ) and also by ELISA ( Supplementary Fig. 4b ). For affinity measurements by microscale thermophoresis (MST), the concentration of the fluorescently labelled transferrin molecule was kept constant at 70 nM and the concentration of the unlabelled titrant, that is, GAPDH was varied from 2 nM to 2 μM; the K D value was estimated to be 160±24 nM ( Fig. 4a ). 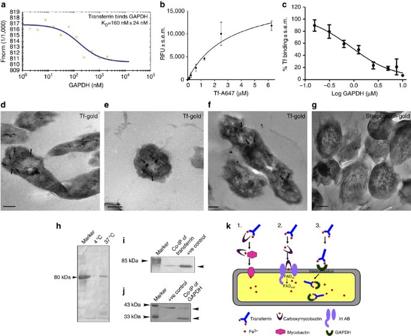Figure 4: Receptor-mediated binding and internalization of transferrin intoM.tbbacilli. (a) The concentration of the NT-647-labelled transferrin was kept constant, whereas the concentration of the rGAPDH was varied. MST analysis was performed with concentrations on thexaxis are plotted in nM. The experiment was repeated multiple times and data from a single experiment are presented (see alsoSupplementary Fig. 4a,b). (b) Saturable binding of Tf-A647 on the surface of intactM.tbH37Ra cells. Data are presented as RFU±s.e.m., experiments were done in duplicates and repeated thrice. Data were fitted to saturation binding curve. (c) Inhibition of transferrin binding in the presence of increasing molar concentrations of rGAPDH. Data are plotted as %Tf binding±s.e.m. versus log GAPDH concentration, experiments were done in duplicates and repeated four times. Data were fitted to inhibitory dose response curve. (d–f). Presence of transferrin-gold particles within the cytoplasm ofM.tbH37Ra cells, after incubation at 37 °C for 1 h. (g) Control cells incubated with Streptavidin-gold conjugate, scale bar, 100 nm. (h) Western blot confirms the presence of biotinylated transferrin in the cytosolic fraction ofM.tbH37Ra cells after internalization at 37 °C as compared with 4 °C. (see alsoSupplementary Fig. 4c). Biotinylated transferrin has been used as molecular weight marker. Transferrin binding proteins are internalized along with transferrin. (i) Capture of internalized biotinylated surface proteins results in pull-down of transferrin, human holo-transferrin was used as positive control (see alsoSupplementary Fig. 6e). (j) Capture of internalized transferrin and detection of associated GAPDH,M.tbcytosol was utilized as the positive control. Prestained molecular weight markers have been run alongside (see alsoSupplementary Fig. 6f). (k) Mechanisms for the uptake of transferrin iron byM.tb.1. Carboxymycobactin acquires transferrin iron, which is then delivered to the bacilli via mycobactin. 2. Carboxymycobactin directly utilizes the high-affinity importer Irt AB to deliver transferrin iron. 3.M.tbsurface proteins promote the internalization and delivery of holo-transferrin independent of siderophores. Figure 4: Receptor-mediated binding and internalization of transferrin into M.tb bacilli. ( a ) The concentration of the NT-647-labelled transferrin was kept constant, whereas the concentration of the rGAPDH was varied. MST analysis was performed with concentrations on the x axis are plotted in nM. The experiment was repeated multiple times and data from a single experiment are presented (see also Supplementary Fig. 4a,b ). ( b ) Saturable binding of Tf-A647 on the surface of intact M.tb H37Ra cells. Data are presented as RFU±s.e.m., experiments were done in duplicates and repeated thrice. Data were fitted to saturation binding curve. ( c ) Inhibition of transferrin binding in the presence of increasing molar concentrations of rGAPDH. Data are plotted as %Tf binding±s.e.m. versus log GAPDH concentration, experiments were done in duplicates and repeated four times. Data were fitted to inhibitory dose response curve. ( d – f ). Presence of transferrin-gold particles within the cytoplasm of M.tb H37Ra cells, after incubation at 37 °C for 1 h. ( g ) Control cells incubated with Streptavidin-gold conjugate, scale bar, 100 nm. ( h ) Western blot confirms the presence of biotinylated transferrin in the cytosolic fraction of M.tb H37Ra cells after internalization at 37 °C as compared with 4 °C. (see also Supplementary Fig. 4c ). Biotinylated transferrin has been used as molecular weight marker. Transferrin binding proteins are internalized along with transferrin. ( i ) Capture of internalized biotinylated surface proteins results in pull-down of transferrin, human holo-transferrin was used as positive control (see also Supplementary Fig. 6e ). ( j ) Capture of internalized transferrin and detection of associated GAPDH, M.tb cytosol was utilized as the positive control. Prestained molecular weight markers have been run alongside (see also Supplementary Fig. 6f ). ( k ) Mechanisms for the uptake of transferrin iron by M.tb. 1. Carboxymycobactin acquires transferrin iron, which is then delivered to the bacilli via mycobactin. 2. Carboxymycobactin directly utilizes the high-affinity importer Irt AB to deliver transferrin iron. 3. M.tb surface proteins promote the internalization and delivery of holo-transferrin independent of siderophores. Full size image Characterization of transferrin binding to M.tb cells Binding of transferrin onto M.tb H37Ra cell surface was concentration dependent and saturable, indicative of the presence of receptor-mediated binding to cells ( Fig. 4b ). The total number of transferrin binding sites was estimated to be 7,136±255 per cell. To evaluate the specificity and the relative importance of GAPDH as a transferrin receptor on M.tb cells, inhibition of transferrin binding to bacilli in the presence of molar excess of rGAPDH was measured. Addition of increasing molar concentrations of rGAPDH resulted in a steady decrease of transferrin binding ( Fig. 4c ) with up to ~80% inhibition of transferrin binding being achieved. Internalization of transferrin and GAPDH After incubation of cells for 1 h at 37 °C, the presence of transferrin-labelled gold particles was observed by TEM in the cytoplasm of M.tb , indicating that transferrin is internalized into cells. Tomography of intact bacteria that had internalized labelled transferrin also clearly revealed the presence of Tf-gold particles within the cytoplasm with practically no particles remaining bound at the surface of the bacilli ( Fig. 4d–f , Supplementary Movie 1 , Supplementary Fig. 7 ). No internalization was evident in controls ( Fig. 4g ). Western blotting of purified cytoplasmic fractions provided further evidence that transferrin is indeed internalized after incubation of cells at 37 °C but not at 4 °C ( Fig. 4h ). These results are in concurrence with those of iron uptake experiments ( Fig. 3f,g ). Transferrin internalization was also similarly confirmed in both M. smegmatis wild-type and M. smegmatis Δesx-3 strains ( Supplementary Fig. 4c ). The internalization of the transferrin-binding protein complex was confirmed by pull-down of surface biotinylated proteins and detection of associated transferrin in the cytosolic fraction ( Fig. 4i , and Supplementary Fig. 6e ). In a reverse experiment, internalized transferrin captured onto Protein-A beads pre-coated with anti-transferrin antibody were observed to co-immunoprecipitate GAPDH ( Fig. 4j , Supplementary Fig 6f ). Internalization of Tf in intracellular bacilli To demonstrate that the interaction of M.tb GAPDH and transferrin is relevant during infection, the trafficking of transferrin was analysed in THP-1 macrophages infected with M.tb H37Ra GAPDH-mCh, M.tb H37Ra mCh, M. smegmatis mCh or M. smegmatis Δesx-3 mCh strains. Transferrin was observed to colocalize to the intracellular bacteria in all strains assessed ( Supplementary Fig. 5a–d ). To determine whether the transferrin is localized within the intracellular bacilli, post infection, cells were first incubated with Tf-A647 to allow internalization. Subsequently, bacilli resident in the phagosome were isolated and treated with pronase to digest any surface-bound transferrin. Bacilli were then analysed for the presence of fluorescence corresponding to Tf-A647. Significantly, the M.tb H37Ra strain expressing GAPDH mCh demonstrated an almost twofold increase of Tf-A647 internalization as compared with control strains ( P < 0.0005 using Student’s t -test; Fig. 5a ). In isolated phagosomal bacilli, fluorescence signals for both GAPDH mCh and Tf-A647 were evident ( Fig. 5b ). The experiment was repeated using transferrin. A pull-down of internalized transferrin from the cytoplasmic fraction of isolated intracellular M.tb H37Ra resulted in the co-immunoprecipitation of M.tb GAPDH ( Fig. 5c , Supplementary Fig. 6g ). Both M. smegmatis wild-type and M. smegmatis Δesx-3 strains demonstrated an internalization of Tf-A647, indicating that uptake of transferrin is independent from siderophore-mediated iron uptake ( Fig. 5d ). This suggests that not only is transferrin transported to the phagosome during infection, but it is also internalized into the bacilli via specific receptors. 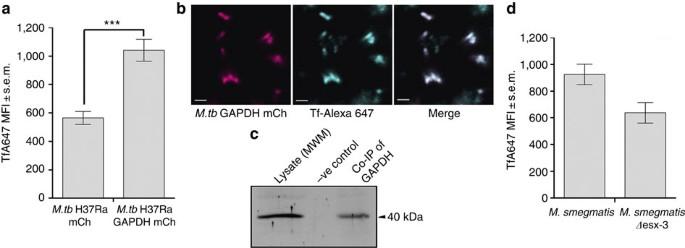Figure 5: Transferrin is localized to and internalized by intraphagosomal bacilli during infection. (a)M.tbGAPDH-mCh isolated from THP-1 macrophages indicate a significantly higher internalization of Tf-A647 as compared with the controlM.tbH37Ra mCh strain. Data are plotted as MFI of 104cells per sample±s.e.m., experiments were repeated thrice(***P<0.0001,n=3) significance was determined using Student’st-test (see alsoSupplementary Fig. 5). (b) Isolated intraphagosomalM.tbH37Ra GAPDH mCh bacteria exhibit colocalization of mCherry and Tf-A647 signals, scale bar, 2 μm. (c) Transferrin internalized by bacilli in phagosomes interacts with mycobacterial GAPDH. THP-1 cells were infected with theM.tbH37Ra strain. Subsequent to internalization of transferrin, bacilli were isolated and cytosolic fractions prepared. The pull-down of transferrin in this fraction resulted in the co-immunoprecipitation of GAPDH as detected by western blotting with α-GAPDH antibody.M.tblysate alone has been run as a positive control (see alsoSupplementary Fig. 6g). (d) BothM. smegmatiswild-type andM. smegmatisΔesx-3 bacilli isolated from the phagosome demonstrate the presence of internalized Tf-A647. Data are plotted as MFI of 104cells per sample±s.e.m., experiments were repeated thrice. Figure 5: Transferrin is localized to and internalized by intraphagosomal bacilli during infection. ( a ) M.tb GAPDH-mCh isolated from THP-1 macrophages indicate a significantly higher internalization of Tf-A647 as compared with the control M.tb H37Ra mCh strain. Data are plotted as MFI of 10 4 cells per sample±s.e.m., experiments were repeated thrice (***P < 0.0001 , n =3) significance was determined using Student’s t -test (see also Supplementary Fig. 5 ). ( b ) Isolated intraphagosomal M.tb H37Ra GAPDH mCh bacteria exhibit colocalization of mCherry and Tf-A647 signals, scale bar, 2 μm. ( c ) Transferrin internalized by bacilli in phagosomes interacts with mycobacterial GAPDH. THP-1 cells were infected with the M.tb H37Ra strain. Subsequent to internalization of transferrin, bacilli were isolated and cytosolic fractions prepared. The pull-down of transferrin in this fraction resulted in the co-immunoprecipitation of GAPDH as detected by western blotting with α-GAPDH antibody. M.tb lysate alone has been run as a positive control (see also Supplementary Fig. 6g ). ( d ) Both M. smegmatis wild-type and M. smegmatis Δesx-3 bacilli isolated from the phagosome demonstrate the presence of internalized Tf-A647. Data are plotted as MFI of 10 4 cells per sample±s.e.m., experiments were repeated thrice. Full size image Despite several studies that suggest trafficking of the iron carrier protein transferrin to the phagosome, relatively little is known as to how iron is withdrawn from these molecules and delivered into the bacteria [12] . Our studies demonstrate for the first time that mycobacterial proteins sequester transferrin at the bacterial surface. Six interacting proteins were identified which included iron-regulated elongation factor tu (Rv0685), L -Lactate dehydrogenase (Rv1872c), acyl-carrier protein desaturase (Rv0824c), the 50S ribosomal proteins L1 (Rv0641), L2 (Rv0704) and glyceraldehyde-3-phosphate dehydrogenase (Rv1436). Of these proteins, homologues of elongation factor tu [36] , L -Lactate dehydrogenase [37] and ribosomal proteins [38] are known to be multifunctional in other organisms while GAPDH is known to be a virulence factor for several pathogens [29] , [30] , [31] , [32] , [33] . GAPDH has also been reported as a transferrin-binding protein in S. aureus and S. epidermidis [21] . In eukaryotes, numerous functions have been attributed to GAPDH including its role as a receptor for transferrin in different cell types and especially in macrophages [26] , [27] , [28] , [39] . Since this molecule is highly conserved across species (~50% identity with human GAPDH), we initially selected GAPDH to further explore the role of this transferrin-binding protein in M.tb . Our results confirmed that GAPDH specifically binds to holo-transferrin rather than apotransferrin, and that its expression on the mycobacterial cell surface is sensitive to iron depletion, as observed for other proteins involved in iron metabolism [2] , [3] , [40] . The presence of GAPDH in cytosol, cell membrane and cell wall fractions of virulent and avirulent strains was confirmed. This observation is in accordance with previous results where it has been identified as a 43.6-kDa culture filtrate protein of M. bovis [41] and as a membrane-associated protein in M.tb H37Rv [42] , [43] , [44] , [45] . The presence of GAPDH and other glycolytic proteins on the surface of several prokaryotes and eukaryotic cells, despite the lack of a distinct secretory signal, has been referred to as ‘nonclassical secretion’ [46] , [47] and a bioinformatics-based analysis of M.tb GAPDH failed to predict any secretion via the sec-dependent or twin arginine translocation system [41] . In the current study, multiple proteins have been identified to interact with transferrin. Using microscale thermophoresis we identified the K D value of GAPDH–Tf interaction to be 160±24 nM. The addition of molar excess of recombinant protein, inhibited transferrin binding onto the cell surface by ~80% indicating that GAPDH is an important component of transferrin receptor-mediated iron uptake in M.tb . For further studies involving GAPDH-mediated transferrin-iron acquisition, strains overexpressing GAPDH were utilized, these clearly demonstrated an enhanced sequestration of transferrin at the cell surface that correlated with an increase of both transferrin binding and iron acquisition. A knockout strain was not utilized as GAPDH has been reported as an essential gene by transposon mutagenesis [48] . We considered a previous report which demonstrates that carboxymycobactins first withdraw transferrin iron, which is then transferred to membrane-bound mycobactins. According to this study, mycobactins are incapable of directly acquiring transferrin iron for the cell [9] . This inference was based on experiments where M.tb cultures were incubated either with ferri-carboxymycobactin or transferrin and iron uptake was evaluated by measuring the amount of ferri-mycobactin. These experiments did not evaluate total cellular uptake of transferrin-bound iron into the cells, which might have occurred by the alternate mechanism described in this study. Supporting the existence of siderophore-independent mechanisms are reports of the recombinant BCG( mbtB )30 strain that was unable to synthesize both mycobactin and carboxymycobactin yet survived in vivo and was able to acquire transferrin iron [14] . In addition, the acquisition of transferrin iron by mycobactins is a relatively slow process; studies have demonstrated that after 24 h of incubation only 30% of mycobactin was converted to Fe-mycobactin [49] . However, the uptake of transferrin iron observed in our experiments was rapid with increased cellular iron levels observed within 6 h for M.tb H37Ra and within 1 h for M. smegmatis strains. Crucially, the M. smegmatis Δesx-3 strain that is unable to utilize mycobactin [35] retained its ability to acquire transferrin iron to levels comparable with that of the wild-type strain. Siderophore synthesis occurs only after culture in iron-free media. In our studies the short pre-incubation (in media lacking iron) and incubation times (with transferrin) coupled with washing steps excludes the possibility that carboxymycobactin or exochelins are synthesized to be present extracellularly for withdrawal of transferrin iron. We then considered the hitherto unreported possibility that transferrin could be internalized into the bacterium as is observed in mammalian cells. Using multiple approaches we unequivocally demonstrate that sequestration of holo-transferrin at the bacterial surface is followed by its internalization into the cytoplasm at 37 °C. Transferrin internalization was detected in M.tb H37Ra (1 h) and M. smegmatis strains including the M. smegmatis Δesx-3 strain within 20 min. In the context of intraphagosomal bacilli, both M.tb and M. avium infected macrophages are known to acquire transferrin and lactoferrin iron by recruiting these host proteins to the phagosome [5] , [6] , [7] , [8] . Interestingly, it is also known that M.tb and M. bovis BCG strains incapable of synthesizing siderophores, survive intracellularly [5] , [14] . Within the first hour of infection, the phagosomal vacuole containing M.tb H37RvO1A siderophore knockout strain acquired more transferrin iron than the wild-type M.tb H37Rv strain [5] . However, 24 h post infection, the mutant strain displayed lower iron levels than the wild type. Survival of the rBCG( mbtB )30 strain also appeared to be independent of siderophores at the early stages of infection in in vivo studies using SCID mice [14] . This suggests that during establishment of infection a rapid siderophore-independent uptake mechanism for transferrin iron may exist. While at later stages, once bacilli sense iron depletion, siderophore-mediated uptake may become the primary route for iron uptake via transferrin [5] . Significantly, five of the six transferrin-binding proteins reported in the current study have been identified as a part of the surface proteome of non-phagocytosed and phagocytosed M. avium [50] and M. smegmatis [51] , although till date, no precise function had been attributed to them. In addition, recent proteomic analysis of M. tuberculosis H37Rv has revealed the presence of all six proteins in the cell wall and membrane fraction [44] , [45] . To understand the relevance of the GAPDH–Tf pathway during infection, colocalization of transferrin to intraphagosomal bacilli was confirmed using a macrophage cell culture model. To establish that transferrin is not merely trafficked to phagosome, but is actively internalized by the bacilli, isolated intraphagosomal bacilli were assessed for the presence of internalized Tf-A647 post infection. GAPDH-overexpressing M.tb demonstrated significantly higher levels of transferrin uptake. In addition, co-immunoprecipitation confirmed the presence of transferrin within the cytosolic fraction of bacilli isolated from macrophages. Based on these results we propose that M.tb can acquire transferrin iron by three mechanisms ( Fig. 4k ). The first is withdrawal of iron by carboxymycobactin, transfer of iron to mycobactin and subsequent intracellular delivery. The second mechanism involves the withdrawal of transferrin iron by carboxymycobactin, and delivery of iron to the bacilli using the high-affinity transporter IrtAB by a mycobactin-independent pathway. Finally, our present studies reveal an additional route for transferrin-iron acquisition that is independent of siderophores and involves the internalization of transferrin by GAPDH and perhaps other identified surface proteins into the bacterium with ferrireductases (present within the cytoplasm) being involved in the removal of iron from transferrin. These findings should also be considered in light of numerous reports that associate high serum iron levels and transferrin-iron saturation with an increased mortality and morbidity due to tuberculosis [16] , [17] , [18] , [19] , [20] . It is possible that extracellular M.tb present in a transferrin-rich environment utilize this pathway for immediate access to iron. With consideration to our recent results as well as previous studies [5] , this mechanism could also be important in the establishment of infection, until such a time that siderophore synthesis and secretion is initiated. A mechanism similar to receptor-mediated endocytosis has only been reported previously in the bacteria Gemmata obscuriglobus [52] . Taken together, this study provides a completely new perspective not only in terms of iron acquisition but also the possibility of receptor-mediated uptake and trafficking that has never previously been reported in M.tb. Mycobacterial strains M.tb H37Ra and M. smegmatis mc 2 155 strains were obtained from microbial-type culture collection, Institute of Microbial Technology (IMTECH), Chandigarh. Mycobacterial strains, M. tuberculosis H37Ra and M. smegmatis mc 2 155 were grown in Middlebrook’s 7H9 broth supplemented with glycerol, OADC and Tween 80 or Middlebrook’s 7H10 agar supplemented with glycerol and OADC at 37 °C. M. smegmatis Δesx-3 strain was a kind gift from Professor E. Rubin, Harvard School of Public Health, USA [35] . Surface binding of Transferrin on M.tb M.tb H37Ra, M. smegmatis wild-type and M. smegmatis Δesx-3 cells were cultured to log phase, 2 × 10 8 cells were used per assay. Cells were washed with phosphate-buffered saline (PBS) and blocked for 1 h at 4 °C with PBS containing 2% BSA. Cells were then incubated with holo-Tf-A647 (Invitrogen; 20 μg per 100 μl of PBS, 1% BSA) alone or in the presence of 200-fold excess unlabelled human holo-transferrin (Sigma) at 4 °C for 2 h. Finally, cells were washed extensively with PBS and fluorescence data of 10 4 cells per assay was acquired using a BD FACS Verse instrument. Experiments were repeated thrice, representative data of one experiment is shown, statistical significance was determined by Student’s t -test. For immunogold labelling, log phase M.tb H37Ra cell pellets were washed with PBS containing 0.2% casein followed by blocking with PBS containing 2% casein at 4 °C for 1 h. To detect transferrin binding, 2 × 10 8 cells were incubated with 20 μg transferrin-gold particles in 100 μl PBS, 0.2% casein for 2 h at 4 °C, particles were prepared as described previously [53] . Cells were fixed in Karnovsky’s fixative for 30 min, followed by two washes with 5 mM NaCl. Finally, cells were resuspended in PBS, placed on carbon-coated grids and viewed in a JEOL 2100 TEM. As a negative control, samples were similarly incubated with streptavidin-gold conjugate (20 nm, Sigma) instead of transferrin. Co-imunoprecipitation of M.tb proteins with transferrin Transferrin-biotin (Sigma, 500 μg) was incubated with 100 μl of streptavidin paramagnetic particles (SAPMPs) (Pierce) for 1 h at 4 °C on a rotospin. Particles were washed with PBS and mixed with 1.5 mg of M.tb H37Rv cell membrane (obtained from BEI Resources, NIAID, USA) for 2 h at 4 °C. After exhaustive washes with PBS, the beads were boiled for 15 min in 30 μl Laemmli sample buffer. To observe the interacting proteins, a 10% SDS–polyacrylamide gel electrophoresis (SDS–PAGE) gel was run and stained with Coomassie blue. Control experiments were carried out with an equivalent amount of biotinylated carbonic anhydrase instead of transferrin. Peptide mass fingerprinting The most prominent bands observed to co-immunoprecipitate with transferrin were in the range of 30–40 kDa, six of these bands were excised from 10% SDS–PAGE stained gels, PMF was carried out at Vimta Labs, Hyderabad, India. Database searching (Swiss-Prot) was restricted to M. tuberculosis complex, and protein identification were performed with MASCOT Software ( http://www.matrixscience.com ), with trypsin plus one missed cleavage, carboxyamidemethylation as a fixed modification and methionine oxidation as a variable modification and a mass tolerance of 0.5 Da for the precursor molecular weight. The criteria to accept a protein hit as a valid identification was multiple tryptic peptide matches to the protein sequence and a significance of P <0.05 (ref. 25 ). Polyclonal antibody against mycobacterial GAPDH A peptide of residues 59–100 from the M.tb H37Rv GAPDH sequence was synthesized for immunization. Rabbits and mice were handled according to the guidelines of Institutional Animal Ethics Committee, National Institute of Pharmaceutical Education and Research (NIPER). Primary immunization of two 12–18-week-old NZW female rabbits was done as described previously [54] . Animals were bled four days after last immunization and serum was prepared. The specificity of the antibody was determined by western blotting against lysates (40 μg per lane) from M.tb H37Rv (positive control), M. smegmatis , Escherichia coli JM109, Saccharomyces cerevisiae , SP2/O.Ag14 (mouse myeloma) and THP-1 (human macrophage cell line). Prestained molecular weight marker (New England Biolabs) was run alongside samples. GAPDH was detected using the α-GAPDH rabbit polyclonal antibody (1:1,000) for 1 h, followed by incubation with goat α-rabbit IgG-HRP for 1 h. Finally, blots were washed and developed with TMB/H 2 O 2 (Bangalore Genei). A polyclonal mouse antibody was similarly raised in 6–8-week-old female Balb/c mice immunized with 50 μg antigen, followed by three boosters. GAPDH enzyme assay of cellular fractions The enzymatic activity of GAPDH was evaluated in cytosol, membrane and cell wall fractions of M.tb H37Rv as described previously using multiple batches of samples obtained from Biodefense and Emerging Infections (BEI) Research Resources Repository [55] . Briefly, 50 μg of M.tb H37Rv samples were added to wells containing 200 μl of assay buffer (50 mM HEPES, 10 mM sodium arsenate and 5 mM EDTA, pH 8.5), 1 mM NAD + and 2 mM G-3-P (Sigma) at 25 °C. Rabbit muscle GAPDH (RM-GAPDH, 400 ng per 200 μl assay buffer; Sigma) was used as a positive control. Enzyme activity was measured as the increase in absorbance at 340 nm due to the formation of NADH at the end of 10 min. For negative controls, assays were carried out with buffer lacking the specific substrate G-3-P, these values were subtracted from the final absorbance. Co-immunoprecipitation of Tf and GAPDH Transferrin-biotin was first mixed with 100 μl of SAPMPs (Pierce) for 1 h at 4 °C on a rotospin. The particles were washed with PBS and incubated with 1–2 mg of protein from cytosol, cell membrane or cell wall fractions of M.tb H37Rv for 2 h at 4 °C. After washing with PBS, particles were resuspended in 30 μl of Laemmli sample buffer, boiled and loaded on a 10% SDS–PAGE gel. As a negative control, SAPMPs were pre-loaded with an unrelated biotinylated protein (carbonic anhydrase) and similarly processed. Captured GAPDH was detected by western blotting using α-GAPDH antibody, as described previously. Prestained molecular weight markers were run with each experiment. FRET analysis of transferrin and GAPDH interaction Log phase cultures of M.tb H37Ra expressing GAPDH mCh or mCh alone were used for analysis. Cells were washed and blocked as for TEM studies and incubated with 20 μg transferrin-Alexa 488 (Tf-A488, Invitrogen) in 100 μl PBS, 1% BSA for 2 h at 4 °C. Samples were fixed in 4% buffered paraformaldehyde for 20 min and FRET analysis was carried out by the acceptor photobleaching method on a Nikon A1R confocal microscope as described previously [26] . The intensities of a total of 12 regions of interest from multiple, randomly selected fields were measured before and after photobleaching. The % intensity change after bleaching was calculated for both acceptor and donor signal. Statistical analysis was done by Student’s t -test. Co-localization of GAPDH and Tf on M.tb cells by TEM M.tb H37Ra GAPDH mCh cells were cultured to log phase, washed and blocked as described earlier for TEM samples. Aliquots of cells were then incubated with either 1:100 polyclonal rabbit α-GAPDH or an equivalent quantity of pre-immune sera for 1 h. Cells were subsequently washed and incubated with a 1:10 α-rabbit IgG 5 nm gold conjugate (Sigma) along with 4 μg Tf-gold per 100 μl PBS, 0.2% caesin for 2 h before fixation in Karnovsky’s fixative for 30 min, all incubations were carried out at 4 °C. Finally washed cells were placed on carbon-coated grids for observation in TEM. Regulation of surface GAPDH and Tf binding on iron depletion M.tb H37Ra cells were grown till early log phase followed by incubation with 150 μM 2,2′-Bipyridyl (Sigma) for 24 h [35] . Controls were maintained in Middlebrooks 7H9 media alone. Cell surface GAPDH expression and transferrin binding on intact cells was determined by ELISA [56] . Briefly, 2 × 10 7 M.tb H37Ra cells per well were incubated overnight at 4 °C in 96-well ELISA plates. Wells were blocked with PBS containing 2% BSA at 4 °C for 2 h followed by three washes with PBS containing 0.05% Tween 20. Plates were incubated with 1:50 polyclonal rabbit α-GAPDH or equivalent pre-immune sera in PBS containing 1% BSA at 4 °C for 2 h. Plates were then incubated with 1:5,000 dilution α-rabbit IgG alkaline phosphatase-conjugated antibody (Sigma) at 4 °C for 2 h and washed. Finally 50 μl per well of substrate solution, that is, 1 mg ml −1 of p -nitrophenylphosphate (Sigma) in substrate buffer (0.001 M MgCl 2 , 0.05 M Na 2 CO 3, pH 9.8) was added to each well. Absorbance was measured at 405 nm after incubation for 1 h at room temperature. Background readings of pre-immune sera controls were subtracted from samples, data are plotted as fold increase as compared with controls. Statistical analysis was done using Student’s t -test, experiments were done in duplicates and repeated thrice ( n =3). To measure transferrin binding, M.tb H37Ra cells were cultured to log phase and 2 × 10 8 cells were used per assay. Cells were washed with PBS and blocked in PBS containing 2% BSA at 4 °C for 1 h. Cells were then incubated with 20 μg of Tf-A647 in 100 μl PBS, 1% BSA at 4 °C for 2 h. Cells were washed and finally resuspended in 200 μl PBS and plated in clear bottom black well plates (Corning). Tf-A647 fluorescence was measured using a Tecan M200 plate reader at excitation 650 nm and emission 668 nm. Background fluorescence of unstained cells was subtracted from all values, data are plotted as fold increase as compared with controls. Statistical analysis was done using Student’s t -test, experiments were done in duplicates and repeated thrice ( n =3). Cell surface enzyme activity M.tb H37Ra, GAPDH mCh and mCh transformants were pelleted and washed with neutral buffer [26] . Cells were then resuspended at a concentration of 1 × 10 8 cells per assay tube in 200 μl assay buffer (pH 8.0) as described earlier. After 30 min of incubation at 25 °C, the OD 340 nm of cell free supernatant was recorded [57] . Measurement of surface GAPDH, Tf and apo-Tf binding on M.tb Cell surface GAPDH expression, transferrin and apotransferrin binding on intact M.tb H37Ra GAPDH-mCh and M.tb H37Ra mCh cells was determined by ELISA, essentially as described in previous experiments [56] . Apotransferrin (Calbiochem) was labelled with Alexa 647 dye (AnaSpec, HiLyte Fluor 647) according to the manufacturer’s protocol. For estimation of surface GAPDH, background readings of pre-immune sera controls were subtracted from samples and data are plotted as Abs 405 nm±s.d., experiments were done in duplicates and repeated thrice ( n =3). Statistical analysis was done using Student’s t -test. Tf-A647 and Apotransferrin-A647 fluorescence was measured as before, background fluorescence of unstained cells were subtracted from all the values, data are plotted as relative fluorescence units (RFU)±s.e.m., experiments were done in duplicates, thrice independently ( n =3). Measurement of transferrin-iron uptake by Tf- 55 Fe M.tb H37Ra mCh and M.tb H37Ra GAPDH-mCh cells were cultured to log phase, 2 × 10 8 cells were used for each assay. Cells were washed twice with Sauton’s media without iron followed by incubation with the same media for 3 h at 37 °C. Cells were then washed and incubated for a further 3 h at 37 °C with media containing 50 μg of Tf- 55 Fe in 100 μl Sauton’s media without iron. Cells were washed thrice with iron-free media, pelleted and resuspended in 3 ml of scintillation fluid. The radioactivity associated with the cell pellet was measured using a β counter (Perkin Elmer), counts were normalized to cell number. M. smegmatis and M. smegmatis Δesx-3 were incubated for 1 h at 37 °C with media containing 50 μg of Tf- 55 Fe and similarly processed. Transferrin-iron uptake by calcein fluorescence quenching Transferrin-mediated iron uptake was assessed by a modification of the calcein-AM quenching assay [58] . Log phase M.tb H37Ra mCh and GAPDH-mCh transformants were washed twice with Sauton’s media lacking iron and staining was performed essentially as described previously [59] . Briefly, 2 × 10 8 cells per assay were incubated with 1 μM calcein-AM (Sigma) at 37 °C for 150 min. Cells were then washed thrice with iron-free Sauton’s media and resuspended in 100 μl of media with or without 50 μg transferrin at 4 °C or 37 °C for 6 h. Finally, cells were washed and fluorescence data from 10,000 cells per sample were acquired, using a Guava Soft Express Pro Flowcytometer. To confirm the sensitivity of the assay, M.tb H37Ra cells were pre-incubated with calcein as described above followed by incubation with Sauton’s media [60] containing ferric ammonium citrate at 4 °C or 37 °C or media without iron. Data are plotted as mean fluorescence intensity (MFI)±s.e.m. of 10 4 cells, experiments were done in duplicates and repeated thrice ( n =3), statistical significance was determined using Student’s t -test. Affinity measurements by Microscale Thermophoresis (MST) Human Holo-transferrin was labelled with a fluorescent dye NT-647 using Monolith NT Protein Labeling Kit RED-NHS as per manufacturer’s instructions. The concentration of the fluorescently labelled transferrin molecule was kept constant at 70 nM and the concentration of the titrant, that is, GAPDH was varied from 2 nM to 2 μM. A serial dilution of the non-labelled titrant GAPDH was prepared using a Tris saline buffer (50 mM Tris, 150 mM NaCl, pH 7.4) containing 0.05% Tween 20. Serial dilutions of the non-labelled GAPDH molecules (10 μl each) were mixed with 10 μl of the fluorescently labelled transferrin molecule. The final sample was loaded into Monolith NT.115 capillaries, followed by analysis with the Monolith NT.115 instrument (Nanotemper) [61] . Determination of cell surface receptor number Log phase M.tb H37Ra cells were washed and blocked in PBS containing 2% BSA at 4 °C for 1 h. Cells were then incubated with increasing concentrations (125 nM–6.25 μM) of Tf-A647 at 4 °C for 2 h. After washing, cells were resuspended in 200 μl PBS and plated in clear bottom black well plates (Corning).Tf-A647 bound at the cell surface was measured using a Tecan M200 multimode reader at excitation and emission wavelengths of 650 and 688 nm, respectively. Background fluorescence of unstained cells was subtracted from all the values, and the data of RFU±s.e.m. of Tf-A647 versus concentration of Tf-A647 were plotted to obtain a saturation curve using Graph Pad Prism Software version 5.01. Receptor number per cell was calculated essentially by the three-tube method [62] , details are provided in Supplementary Methods . Inhibition of transferrin-GAPDH interaction by rGAPDH To assess specificity of interaction on cells, binding of transferrin was measured after pre-blocking with recombinant M.tb GAPDH. Briefly, 2.5 μM (20 μg) of Tf-A647 was pre-incubated with increasing amounts (0.0625 to fourfold) of rGAPDH for 1 h at 4 °C. Bacilli were then incubated with the mixture for 2 h at 4 °C. Tf-A647 fluorescence was measured using a Tecan M200 plate reader at excitation 650 nm and emission 668 nm. Background fluorescence of unstained cells was subtracted from all the values. Data are plotted as % transferrin binding±s.e.m. versus log GAPDH concentration, experiments were done in duplicates and repeated four times ( n =4), values of cells stained with Tf-A647 alone were considered as 100% binding. Transferrin-gold internalization by M.tb using TEM Log phase M.tb H37Ra cells ~6 × 10 9 cells, were washed twice with Sauton’s media without iron and incubated with transferrin-gold (15 μg per 150 μl of media) for 1 h at 37 °C. After washing with the same medium, cells were fixed and embedded in epoxy resin. Ultrathin sections were stained with 2% uranyl acetate and examined in TEM. As a control, cells were treated with Streptavidin-gold conjugate and processed similarly. For intact cell analysis, a suspension of fixed bacteria was applied to a carbon-coated grid and isolated bacilli labelled with Tf-gold were subjected to tomographic analysis using the JEOLTEMOGRAPHY system. A±70° tilt series was acquired at 1° intervals. After alignment of the image series a weighted face back projection was constructed using the JEOL composer software. Internalization of Transferrin and GAPDH by M.tb Log phase M.tb H37Ra cells (~1.5 × 10 10 ) were washed twice with Sauton’s media without iron and incubated with 100 μg of biotinylated transferrin for 1 h at 37 °C. Subsequently cells were washed thrice and resuspended in lysis buffer. The cytosolic fraction was isolated as described earlier, mixed with 100 μl of SAPMPs and incubated for 1 h on a rotospin. Particles were washed extensively with PBS and boiled in 30 μl of Laemmli sample buffer. As a negative control, cells were incubated with biotinylated transferrin at 4 °C and were processed similarly. Captured transferrin-biotin was detected by western blotting using 1:1,000 dilution of α-transferrin rabbit polyclonal antibody (Abcam) followed by incubation with goat α-rabbit IgG-HRP and developed with TMB/H 2 O 2 (Bangalore Genei, India). Biotinylated transferrin (Sigma) was used as molecular weight marker. Co-trafficking of transferrin and M.tb surface proteins Cell surface proteins of M.tb H37Ra cells, (~1.5 × 10 10 per assay) were labelled using Sulfo-NHS-Biotin (Pierce) as per manufacturer’s instructions. Cells were then incubated with 100 μg of transferrin at 37 °C for 30 min to allow for internalization. After three washes cells were resuspended in lysis buffer. The cytosolic fraction was isolated as described previously [63] and incubated with 100 μl of SAPMPs for 1 h on a rotospin to capture internalized biotinylated proteins. Finally, beads were resuspended in 30 μl of Laemmli sample buffer, boiled for 15 min and loaded on a 10% SDS–PAGE. Transferrin associated with internalized surface proteins was detected by western blotting as described previously. To confirm our results a reverse co-immunoprecipitation was also performed. Internalized transferrin was captured using 100 μl Protein-A paramagnetic particles (ThermoScientific) pre-incubated with 50 μg rabbit α-transferrin. Transferrin-associated GAPDH was detected by western blotting using α-GAPDH mouse polyclonal antibody at a dilution of 1:1,000. Trafficking of transferrin to intracellular bacilli The human macrophage cell line THP-1 was utilized as an infection model, essentially as described earlier [64] . In brief, to study trafficking of transferrin to bacteria resident within macrophages, THP-1 cells (2 × 10 5 per assay) were activated with 25 ng ml −1 PMA (Sigma) for 24 h followed by resting for additional 24 h. Cells were then shifted to antibiotic-free RPMI media containing 10% fetal calf serum. Infection was done at a ratio of 1:40 (THP-1:bacteria) using log phase cultures of M. smegmatis mCh, M. smegmatis Δesx-3 mCh , M.tb H37Ra mCh or M.tb H37Ra GAPDH-mCh. After 6 h, cells were washed with serum-free media (SFM) to remove non-phagocytosed bacteria. A second wash with SFM was carried out after 24 h of infection and residual transferrin in cells was depleted by incubation in SFM for 1 h at 37 °C [65] . Cells were then washed with SFM and cells were incubated with 20 μg of Tf-A647or Tf-A488 in 100 μl SFM media at 4 °C for 1 h. Subsequently, uptake of bound transferrin was done at 37 °C, 5% CO 2 for 1 h, followed by washes with SFM. Finally cells were fixed with 1% paraformaldehyde for 30 min and imaged on Nikon A1R confocal microscope using a × 63 oil immersion objective and an aperture of 1 airy unit. Transferrin internalization by intraphagosomal mycobacteria THP-1 cells were infected with M.tb H37Ra GAPDH-mCh, M.tb H37Ra mCh, M. smegmatis mCh or M. smegmatis Δesx-3 mCh bacteria as described for microscopy experiments. Post infection, cells were washed with SFM, and ~3 × 10 6 cells were incubated with 50 μg of Tf-A647 in 1.0 ml of buffer for 1 h at 4 °C. Subsequently cells were shifted to 37 °C for 1 h to allow for internalization of bound transferrin. After thorough washing with SFM, intraphagosomal bacilli were isolated from macrophages essentially as described previously [7] . Briefly, cells were lysed with SFM containing 0.1% SDS, 1,000 units per ml DNase followed by centrifugation at 10,000 g for 10 min. Bacteria were then washed thoroughly with 0.01% SDS solution in SFM and incubated with 0.1% pronase for 15 min at 4 °C to remove any remaining surface-bound Tf-A647 (ref. 40 ). Isolated bacteria were analysed using a BD FACS Aria instrument, 10 4 bacterial cells gated for mCherry expression were analysed for the uptake of Tf-A647. Data are presented as MFI of 10 4 cells±s.e.m. for Tf-A647, experiments were repeated thrice ( n =3). Samples were also fixed with 1% paraformaldehyde for 30 min and imaged on Nikon A1R confocal microscope using a × 100 Plan-Apo objective and 1 airy unit aperture to determine colocalization of both signals in isolated bacilli. Interaction of GAPDH and Tf within intraphagosomal M.tb THP-1 cells were infected with M.tb H37Ra, washed with SFM, and ~1 × 10 8 harvested cells were incubated with 1.0 mg of human transferrin in 1 ml of buffer for 1 h at 4 °C. Subsequently cells were incubated at 37 °C, 5% CO 2 for 1 h to allow uptake of bound transferrin. Intraphagosomal bacilli were isolated as described earlier [7] and cytosolic fraction was prepared as described for M.tb H37Ra cells ( Supplementary Methods ) The fraction was incubated with rabbit α-Tf antibody immobilized on goat α-rabbit IgG magna beads (Pierce) overnight at 4 °C on rotamixer. Particles were washed extensively and boiled in Laemmli sample buffer. As a negative control, lysate was incubated with rabbit IgG immobilized on goat α-rabbit IgG magna beads. Transferrin-associated GAPDH was detected by western blotting using α-GAPDH mouse polyclonal antibody at a dilution of 1:1,000 using Luminata Forte (Millipore) as substrate according to manufacturer’s instructions, and scanned on Image Quant (GE Healthcare). How to cite this article: Boradia, V. M. et al. Mycobacterium tuberculosis acquires iron by cell-surface sequestration and internalization of human holo-transferrin. Nat. Commun. 5:4730 doi: 10.1038/ncomms5730 (2014).